Dawn–dusk asymmetry in the Kelvin–Helmholtz instability at Mercury The NASA MErcury Surface, Space ENvironment, GEochemistry and Ranging (MESSENGER) spacecraft entered orbital phase around Mercury on 18 March 2011. A surprising consistent feature in the data returned is large-scale vortices that form exclusively on the dusk side of the magnetosphere. Here we present global kinetic hybrid simulations that explain these observations. It is shown that vortices are excited by a Kelvin–Helmholtz instability near the subsolar point, which grows convectively along the dusk-side magnetopause. Virtual time series along a track approximating a flyby of the MESSENGER show correspondence with the satellite data; the data contain sawtooth oscillations in plasma density, flow and magnetic field, and exhibit the observed dawn–dusk asymmetry. It is shown that asymmetry between dawn and dusk at Mercury is controlled by the finite gyroradius of ions and by convection electric fields. Mercury’s magnetosphere offers a natural laboratory for studying plasma regimes not present in other planetary magnetospheres or the laboratory. Mercury is the closest planet to the Sun, with an orbital radius that varies between 0.309–0.469 AU over a Mercury year (88 Earth days). It has a dipole-like magnetic field similar to Earth, but its dipole moment is smaller, in the range of 195±10 nT ( [1] ). Mercury is smaller than Earth at a radius R M of 2,439 km (0.38 of the Earth’s radii). Its proximity to the Sun means it is strongly affected [2] by the solar wind, which creates a planetary magnetosphere with a size that is about 5% that of the Earth’s magnetosphere. The density of solar wind particles and the strength of the Sun’s magnetic field (IMF) are about an order of magnitude higher at Mercury. This means that the subsolar magnetopause (MP) stand-off distance is quite close to the surface of the planet, at a distance between 1.3 and 2.1 R M ( [3] ), depending on the parameters of the solar wind. Physical processes at Mercury are much more dynamic [4] (timescales of seconds) because of the relatively high Alfvén speed in the solar wind at the orbit of the planet. Before orbit insertion on 18 March 2011, the NASA MESSENGER (MErcury Surface, Space ENvironment, GEochemistry and Ranging) spacecraft [5] performed three [1] , [6] , [7] nearly equatorial flybys. During the third flyby on 29 September 2009, MESSENGER recorded multiple MP crossings that were interpreted as signatures of the Kelvin–Helmholtz instability (KHI) [8] . The KHI is of interest, because it has a strong role in controlling mass and energy transport throughout Mercury’s as well as the Earth’s [9] magnetosphere. The observations [10] , [11] reveal that the KH waves are routinely present with a source region that is close to the subsolar point along the post-noon MP. The KHI also produces disturbances over a large portion of the dayside magnetosphere [11] . It is these observations that we attempt to explain here. It is demonstrated that Mercury’s magnetic environment is dominated by kinetic-scale plasma dynamics that differentiate it from processes occurring in other planetary magnetospheres. The methodology used to study the solar wind interaction with Mercury’s magnetic field is large-scale hybrid kinetic particle simulations [12] . The kinetic approach satisfies the requirement to resolve the finite gyroradius [13] of solar wind particles at Mercury, and provides synthetic particle and magnetic field data that can be compared directly with spacecraft observations. An important aspect of this comparison is that synthetic data contains statistical fluctuations related to how many particles are included in the simulation, whereas spacecraft data is limited by the characteristics of the instrument used to collect data, and the random fluctuations in the quantities being sampled. The statistical fluctuations in simulated data allow instabilities to form spontaneously out of noise that approximates that of the real system. The global hybrid kinetic simulations described below show general agreement with MESSENGER observations, which suggest that the KHI is initiated slightly duskward of the subsolar point, where the plasma flow is still accelerating tailward. This is supported by a simplified analysis of the ideal magnetohydrodynamic (MHD) instability condition for the KHI. The simulations also reveal that as vortices move along the dusk flank, they continue to grow convectively within the bulk flow. MESSENGER spacecraft observations of the KHI at Mercury On 29 September 2009, MESSENGER was on an in-bound dusk-to-dawn trajectory in the nightside equatorial magnetosphere, and had its first crossing of the MP at around 21:27:10 MLT. The spacecraft MAG instrument [14] recorded four sawtooth patterns [8] , [15] in the magnetic field in the intervening period from 21:28:10 to 21:29:50 MLT, during which time the MESSENGER was at a radial distance of roughly 3 R M (7,320 km), and slightly tailward of the dusk side flank. The sawtooth oscillations observed by the spacecraft were interpreted by the MESSENGER team scientists as non-linear stage of the KHI [10] . The IMF orientation in the magnetosheath before these sawtooth oscillations varied from southward to northward [8] , but in the majority of cases where the KHI is observed the IMF is strongly northward [11] . This configuration where the IMF is parallel to the planetary magnetic field in the MP is favourable for the KHI along the equatorial magnetospheric flanks [16] . The 29-September and subsequent observations show a clear asymmetry in the KHI in favour of dusk [11] , which will be explained through consideration of asymmetries in the forces acting on the ions at dusk and dawn. Asymmetry in the KHI at Mercury A hybrid kinetic (particle ions and massless fluid electrons) computer model of the solar wind interaction with Mercury is used. The procedure and algorithm upon which the model is based is detailed in Matthews [17] . The magnetosphere is assumed to be two-dimensional and oriented to lie in the equatorial plane of the planetary orbit of Mercury about the Sun. This approximation corresponds to a planet that is topologically a long cylinder with its axis perpendicular to the Sun–Mercury line in the equatorial plane. The distribution function of protons is initially Maxwellian and constructed using 120 particles in each numerical cell of rectangular size Δ x =0.3 c / ω p (9.7 km). Here is the proton plasma frequency, c is the speed of light, e is the electron charge, ɛ 0 is the vacuum permittivity, and n p and m p are the proton density and mass, respectively. The size of the rectangular simulation domain is L x × L y ∼ 750 2 c / ω p (24,000 2 km) and the time step for advancing particle positions is 0.008 (4.2 ms), where Ω p = eB / m p is the proton gyro frequency. The IMF and solar wind velocity take values of 20 nT and 300 km s −1 , respectively [18] . The boundary conditions are as described in Trávníček [12] . The only difference is that particles hitting the surface of the planet suffer specular reflection, and there is no injection from the surface. The planetary field is dipolar [1] at the start of the simulation, with a dipole moment of 195 nT . A limitation set by computer resources is that the simulated planet is one-third the size of the real system. The stand-off (bow-shock) distance of the solar wind from the surface, and solar wind velocities, are the same as the real system, but timescales are three times faster because of the scale difference between the simulated and actual planetary magnetosphere. Consequences of this are discussed later in the paper. KHI at Mercury The KHI is driven by velocity shear and favours an orientation of the IMF that is parallel to the planetary magnetic field in the equatorial magnetosphere. At Earth, the instability is typically observed on the low-latitude magnetospheric flanks [19] , where fast-flowing plasma in the magnetosheath transitions to slow-moving less-dense plasma earthward of the MP. The amplitude of KHI waves at Earth is reported to be in the range of 30–50 nT ( [20] ), whereas amplitudes at Mercury are in excess of 40 nT ( [8] , [11] ). Mercury is also more dynamic, with the KHI characteristic timescales in the range of seconds [8] compared with minutes at Earth. Finite ion gyroradius effects have a more important role at Mercury because of the large difference in size of the respective magnetospheres, and the fact that the ion gyroradius at Mercury can be comparable to the size of the planet. This is important because the simulations reveal that the finite gyroradius of magnetosheath ions and the convection electric field parallel to the velocity shear gradient at dawn broaden the shear layer in which vortices start to form. This lowers the growth rate and is consistent with results of 2.5 D particle-in-cell simulations by Nakamura et al . [13] The opposite conditions apply at dusk, which is a factor in explaining why the KHI preferentially occurs at dusk. 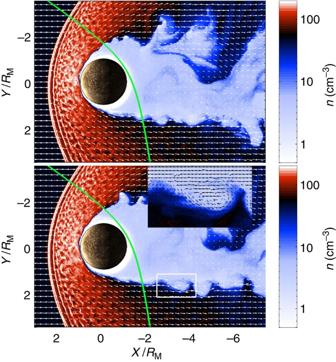Figure 1: Ion density in the equatorial plane of Mercury’s magnetosphere. The ion density obtained from the computer model is shown on a logarithmic scale in the units cm−3together with velocity vectors (represented by arrows), and for different timestΩp=125 and 135, respectively. The magnitude of the upstream vectors corresponds to a velocity of 300 km s−1. The small number of velocity vectors is shown to make the vortices visible. The inset window shows a detail of a single vortex with velocity vectors in the frame of the solar wind. The solid line represents the trajectory of the third flyby of MESSENGER on 29 September 2009. Figure 1 shows two instances of time (ten gyroperiods apart) in the simulated evolution of plasma density around Mercury. The full animation of the density evolution is provided in Supplementary Movie 1 , which shows clearly that the KHI is initiated close to noon and that it grows convectively along the flank MP. The IMF is northward with solar wind flowing from the left, compressing the dayside magnetosphere and moving it towards the planet. Material that accumulates in the vicinity of the subsolar point escapes to the nightside through a relatively small opening or nozzle. This causes plasma to be accelerated tailward starting at low velocity, thus forming a velocity shear between the escaping plasma and slower-moving less-dense plasma adjacent to the planet. The relatively slow-moving plasma in the vicinity of the subsolar point is unstable and evolves through the KHI on the dusk-side magnetospheric flank into large-scale vortical structures that move with the direction of the bulk flow. It is the initiation and growth of these vortical structures that we would like to explain. Figure 1: Ion density in the equatorial plane of Mercury’s magnetosphere. The ion density obtained from the computer model is shown on a logarithmic scale in the units cm −3 together with velocity vectors (represented by arrows), and for different times t Ω p =125 and 135, respectively. The magnitude of the upstream vectors corresponds to a velocity of 300 km s −1 . The small number of velocity vectors is shown to make the vortices visible. The inset window shows a detail of a single vortex with velocity vectors in the frame of the solar wind. The solid line represents the trajectory of the third flyby of MESSENGER on 29 September 2009. Full size image To understand the evolution of the KHI at Mercury, it is informative to consider what plasma conditions affect the instability growth rate. A simple approximation to the growth rate of the KHI for a step-like change in the plasma flow velocity can be obtained from ideal MHD in the incompressible gas limit [21] . This yields a threshold condition for the KHI, which is defined by In this expression, subscripts 1 and 2 denote quantities on either side of the velocity jump, which is regarded as a boundary of zero thickness. The quantities n and v A denote number density and Alfven velocity, respectively; k and v 0 correspond to the KHI wave vector and jump in plasma streaming velocity, respectively. To identify the jump in velocity, the velocity jump is monitored in the y direction, assuming a finite thickness Δ that corresponds to conditions for maximum growth of the KHI defined by Miura and Pritchett [22] , that is, k Δ ∼ 0.8. Here k is defined by the wavelength of vortices in the simulations. Assuming k parallel to v 0 , the magnetospheric regions where the threshold condition is exceeded are indicated by the green lines in Fig. 2 . The post-noon MP extending from the dayside to the distant magnetotail (10 R M ) supports laminar-type flow. This implies that the KHI initiated on the dusk magnetospheric flank is able to grow convectively into large-scale vortices. The dawn flank, on the other hand, exhibits only sporadic pockets of unstable growth and lacks the coherence that is necessary for the KHI to grow convectively with the solar wind flow over several cycles. 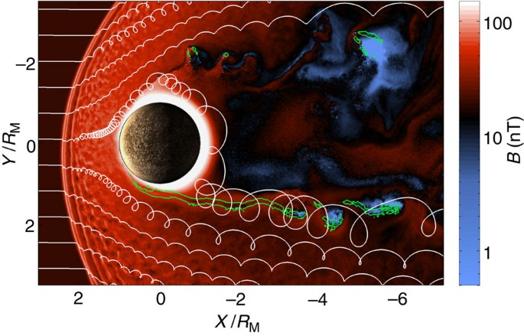Figure 2: Magnetic-field magnitude in the equatorial plane of Mercury’s magnetosphere. The magnitude of the magnetic fieldBat timetΩp=135 is represented by a logarithmic colour scale in the units of nT. Overplotted are trajectories of particles traced from the solar wind as they interact with the magnetic field of the planet. The green curves extending tailward along the dawn (Y∼−1.5) and dusk (Y∼1.5) magnetopause visualize regions most unstable to the KHI. The asymmetry of the unstable regions favours a KHI along dusk. The flow is laminar in the region where the KHI forms, because the convection electric fieldEyis anti-parallel to the velocity-shear gradient. This acts to sustain the gradient by preventing drift of the ions out of the shear layer. Figure 2: Magnetic-field magnitude in the equatorial plane of Mercury’s magnetosphere. The magnitude of the magnetic field B at time t Ω p =135 is represented by a logarithmic colour scale in the units of nT. Overplotted are trajectories of particles traced from the solar wind as they interact with the magnetic field of the planet. The green curves extending tailward along the dawn ( Y ∼ −1.5) and dusk ( Y ∼ 1.5) magnetopause visualize regions most unstable to the KHI. The asymmetry of the unstable regions favours a KHI along dusk. The flow is laminar in the region where the KHI forms, because the convection electric field E y is anti-parallel to the velocity-shear gradient. This acts to sustain the gradient by preventing drift of the ions out of the shear layer. Full size image Figure 2 shows the magnitude of the magnetic field around the planet and trajectories of test particle ions that have kinetic energies equal to the solar wind flow kinetic energy per ion. Although plasma is diverted around the dayside boundary in the expected manner, the particle trajectories show that it penetrates significantly across the bow shock. The ion trajectories in Fig. 2 also show that the gyroradius is comparable with the width of the simple ideal MHD unstable region marked in green on the figure, which confirms that kinetic effects are important in the evolution of the KHI at Mercury. Analysis of the density in Fig. 1 also reveals that with the exception of magnetosheath gradients, the average plasma density and density gradient are larger across most of the dawn-side magnetosphere. This is because the bow-shock location along dawn is moved inward more than at dusk. 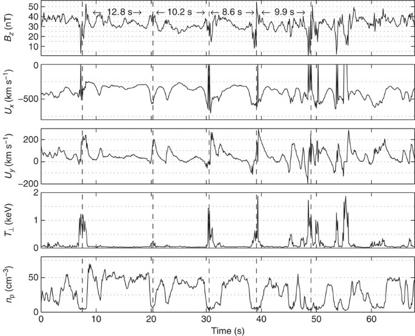Figure 3: Virtual flyby through simulated data. A virtual flyby through synthetic data at locationX,Y=(−2.03, 1.74)RMof theBzcomponent of the magnetic field; bulk flow velocityUx,Uy; perpendicular proton temperatureT⊥; and proton densitynp. The figure is based on a coordinate system in which thexaxis points from Mercury to the Sun; thezaxis is along the dipole moment of the planet; theyaxis completes the right-hand system. Vertical dashed lines represent boundaries of KH vortices as they pass over the virtual satellite. A sawtooth pattern inBzis typical for KH observations. Figure 3 shows synthetic time series ( B z , U x , U y , T ⊥ , n p ) obtained from the simulation. The time series are extracted at a location on the dusk MP where forming of KHI vortices are observed, that, close to the trajectory of the third flyby illustrated by the solid line in Fig. 1 . In the synthetic time series, there are obvious regular sawtooth patterns in the density and similar features in the x -component bulk velocity. The periodicity is on the order of 8–13 s, and is a consequence of the MP boundary sweeping back and forth across the spacecraft as KHI waves move past it. The amplitude of the magnetic perturbations in the first panel of Fig. 3 is on the order of 15–20 nT, whereas the transverse y -component velocity is about 100 km s −1 . The bottom two panels of Fig. 3 show, respectively, MP crossings of high temperature, low-density magnetospheric plasma with low temperature and high-density magnetosheath plasma. Taking into account the one-third scale difference between the modelled and real magnetosphere, these values compare favourably with those reported by MESSENGER. The perpendicular components of the magnetic field perturbations B x and B y are not shown, because the IMF is purely northward in the simulation and is performed in the equatorial plane. Although the pattern of magnetic sawtooth oscillations is similar to that of the velocity perturbations, their amplitude is very small because of the assumed geometry. Figure 3: Virtual flyby through simulated data. A virtual flyby through synthetic data at location X , Y =(−2.03, 1.74) R M of the B z component of the magnetic field; bulk flow velocity U x , U y ; perpendicular proton temperature T ⊥ ; and proton density n p . The figure is based on a coordinate system in which the x axis points from Mercury to the Sun; the z axis is along the dipole moment of the planet; the y axis completes the right-hand system. Vertical dashed lines represent boundaries of KH vortices as they pass over the virtual satellite. A sawtooth pattern in B z is typical for KH observations. Full size image The computer simulation results discussed above reproduce important aspects of the KHI observed by MESSENGER. The asymmetry of the KHI and its preference for the dusk-side flank is shown to be a consequence of asymmetry in dawn and dusk particle motions. On the dusk side of Mercury’s magnetosphere, the convection electric field E y is anti-parallel to the magnetosheath velocity shear gradient and acts to maintain it. This maintains laminar flow at dusk and allows the KHI to grow convectively in the tailward direction. The direction of the convection electric field E y acting parallel to the velocity shear gradient reinforces outward plasma motion at dawn, which leads to broadening of the region in which vortices try to form. Although the KHI is not excluded from the dawn flank, the expectation is that conditions resulting in instability should be less common around dawn. The possibility of an asymmetry in the KHI at Earth also exists, but the evidence is not conclusive. For example, toroidal mode plasma waves on the dawn side of the magnetosphere, as reported by Anderson et al . [23] and Takahashi et al . [24] , have been attributed to the KHI. On the other hand, Taylor et al . [25] have suggested that the KHI is more prevalent around dusk, which is in agreement with observations of Mercury. Global simulations similar to those performed by Claudpierre et al . [26] , but incorporating northward (rather than southward), IMF can potentially answer questions about asymmetry at Earth. On the dawn flank at Mercury, the dynamics of the plasma is such that plasma bubbles form in a manner that is suggestive of a Rayleigh–Taylor-like instability. Such a possibility has been considered by Gratton et al . [27] , but for the solar wind interaction with Earth’s geomagnetic field. A potential contribution to the onset of the KHI that we have not considered arises due to the finite gyroradius of ions in the vicinity of the subsolar point, where shear in the diamagnetic drift velocity v di =( ρ Ω ci B 0 ) −1 B 0 × ∇ P i can be unstable to the KHI [28] . Another important aspect of Mercury’s magnetosphere that we have not considered is the presence of heavy ions. It has been suggested [10] that increased mass loading will enhance the KHI along the dusk flank and create a barrier to the KHI along the dawn flank. The simulations reported here suggest that vortices can form in the absence of heavy ions. It can be concluded that the small scale of Mercury’s magnetosphere in comparison with Earth reveals important differences that will be interesting to assess in the context of other planetary magnetospheres influenced by kinetic scale plasma physics. How to cite this article: Paral, J. and Rankin, R. Dawn–dusk asymmetry in the Kelvin–Helmholtz instability at Mercury. Nat. Commun . 4:1645 doi: 10.1038/ncomms2676 (2013).